A design strategy for the hierarchical fabrication of colloidal hybrid mesostructures Advances in nanotechnology depend upon expanding the ability to create new and complex materials with well-defined multidimensional mesoscale structures. The creation of hybrid hierarchical structures by combining colloidal organic and inorganic building blocks remains a challenge due to the difficulty in preparing organic structural units of precise size and shape. Here we describe a design strategy to generate controlled hierarchical organic–inorganic hybrid architectures by multistep bottom-up self-assembly. Starting with a suspension of large inorganic nanoparticles, we anchor uniform block copolymer crystallites onto the nanoparticle surface. These colloidally stable multi-component particles can initiate the living growth of uniform cylindrical micelles from their surface, leading to three-dimensional architectures. Structures of greater complexity can be obtained by extending the micelles via addition of a second core-crystalline block copolymer. This controlled growth of polymer micelles from the surface of inorganic particles opens the door to the construction of previously inaccessible colloidal organic–inorganic hybrid structures. Nature uses a hierarchy of self-assembly steps to construct functional hybrid structures from inorganic and organic building blocks. Laboratory-based synthetic approaches are now beginning to reach similar levels of exquisite control in the creation of nanoscale and mesoscale architectures [1] , [2] , [3] , [4] , [5] , using well-defined nanomaterials as building blocks. For example, a variety of supramolecular structures have been formed through the secondary association of various organic building blocks [6] including block copolymer (BCP) micelles [7] , [8] , [9] , [10] , [11] , [12] . Higher order structures have also been formed by the self-assembly of inorganic nanoparticles (NPs), including particles with different but complementary shapes, and rod-like particles coated at the ends with DNA or synthetic polymers [13] , [14] , [15] , [16] , [17] . Other types of structures have been generated using BCP micelles, viruses or other scaffolds as templates for decoration with small inorganic NPs [13] , [18] . Although these inorganic NPs add a level of hierarchy to the structure and can have an important functional role (optical, catalytic), they are too small to serve as building blocks for the construction of higher order structures. In contrast, there are only rare examples of colloidal mesoscale structures that combine self-assembled organic building blocks and large inorganic NPs, particularly with the inorganic NP as the central structural unit [19] , [20] . One example that we are aware of consists of DNA origami assemblies attached to a central gold NP, forming ‘core-satellite’ architectures with smaller gold NPs at the periphery. Beautiful as these structures are, the size is limited by the dimensions of the DNA origami and the solvent is restricted to water. It would be a major step forward to enlarge the spectrum of accessible structures, over a larger range of sizes, using a broader variety of organic building blocks, particularly BCP micelles. There are multiple advantages of using BCP micelles as building blocks. Many different BCPs are available, with different chemistries and different functionalities for the core-forming and corona-forming blocks. They can self-assemble in a variety of different selective solvents to form specific morphologies. One can chemically post-modify the corona block of a micelle without altering the properties of its core. Finally, this library of BCPs would offer different ways to anchor the micelles to the surfaces of inorganic particles. This would enable the construction of previously inaccessible colloidal organic–inorganic hybrid mesostructures. We address this challenge via a multistep, bottom-up self-assembly approach to grow uniform cylindrical BCP micelles from the surface of a large inorganic NP as the structural foundation stone. To ensure a high level of structural control over each step of sample preparation, we focus on the fabrication of hybrid hierarchical structures that are colloidally stable during the entire self-assembly procedure. Our examples employ uniform spherical or rod-like inorganic NPs, but our methodology can be applied to central structural units of any size and shape. Then, in a selective solvent, we attach short fragments of a carefully designed core-crystalline BCP micelle. The core polymer is chosen for its ability to initiate crystallization-driven self-assembly (CDSA) of cylindrical BCP micelles when unimer is added to the solution, and the corona must provide strong adhesion to the surface of the inorganic particle. Many BCPs consisting of a long soluble block attached to a shorter crystallizable block [21] are potential candidates for this approach. While CDSA has been reported for BCPs with poly(3-hexylthiophene) [22] , polylactide [23] , polycaprolactone [24] and polyethylene [25] as the crystallizable block, one has the greatest control over this kind of seeded growth for polyferrocenylsilane (PFS) BCPs. Under appropriately chosen self-assembly conditions, all of the added unimer of a PFS BCP grow off the ends of the crystallite seeds in the sample, and uniform elongated structures can be formed [26] , [27] , [28] , [29] , [30] , [31] . The ‘living’ nature of micelle elongation by CDSA thus becomes a tool to control the morphological homogeneity of the structure. Preparation of sunflower-like assemblies To develop our strategy, we began with the fact that a silica surface is rich in Si-OH groups that can form hydrogen bonds in a cooperative way with poly(2-vinylpyridine) (P2VP). Thus, we selected PFS 30 - b -P2VP 300 (the subscripts refer to the number average degrees of polymerization) as the BCP and 250nm diameter silica NPs (SiO 2 NPs, Supplementary Fig. 1 ) as our initial foundation stone. Long cylindrical micelles of PFS 30 - b -P2VP 300 in 2-propanol (2-PrOH) ( Supplementary Fig. 2a ) were prepared as described previously [32] and subjected to mild sonication to obtain a suspension of seed crystallite micelles ( Supplementary Fig. 2b ), characterized by a number average length L n =60 nm (PDI TEM = L w / L n =1.09) uniform in width (number average width, W n =19 nm, PDI TEM =1.03). An aliquot of these crystallites was added to a suspension of the SiO 2 NPs and allowed to age for 24 h. Transmission electron microscopy (TEM) images of this sample are shown in Fig. 1a and Supplementary Fig. 3 . The excess of crystallites present in the solution could be removed by sedimentation and redispersion in fresh 2-PrOH solvent ( Fig. 1b and Supplementary Fig. 4 ). It is important to note that the seed-coated SiO 2 NPs are colloidally stable. They can be submitted to several cycles of centrifugation/redispersion and can be stored for many days, without showing irreversible aggregation. This approach is different from the kinetic trapping of transient PFS homopolymer suspensions by PFS BCP reported recently [33] , where one has only a narrow time window for generating multiarmed structures. The TEM image in the inset of Fig. 1b shows that the crystallites adsorbed to the surface of the silica, adding a layer ~\n30 nm thick. Analysis of the seed-coated SiO 2 NPs by energy-dispersive X-ray (EDX, Supplementary Fig. 5 ) shows strong signals of iron and nitrogen. We refer to these seed-coated NPs both as 1b and as seeds@SiO 2 NPs. To use these NPs as substrates for seeded growth, we added an aliquot of PFS 30 - b -P2VP 300 in tetrahydrofuran (THF) to a suspension of seed-coated SiO 2 NPs in 2-PrOH. After brief swirling, the mixture was set aside to age for 24 h. In this way, the sunflower-like structures ( 1c ) as seen in Fig. 1c and Supplementary Fig. 6 were obtained. This result demonstrates that the PFS 30 - b -P2VP 300 crystallites attached to the NP surface are effective nucleating agents for micelle growth. Because of the large dark circular core seen in the TEM images, we refer to these structures as ‘sunflower’ assemblies. 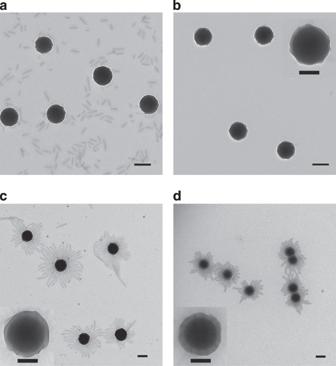Figure 1: Preparation of sunflower-like assemblies through seeded growth and self-seeding. (a) TEM image of a mixture of SiO2NPs and excess PFS30-b-P2VP300seeds prepared in 2-PrOH and aged for 24 h. (b) TEM image of the seed-coated SiO2NPs after removal of excess seeds by sedimentation–resuspension in 2-PrOH. The inset shows a single seed-coated SiO2NP at higher magnification. (c) TEM image of sunflower hybrid assemblies prepared by addition of PFS30-b-P2VP300in THF (15 μl, 10 mg ml−1) to 2-propanol (1 ml) containing seed-coated SiO2NPs (0.5 mg ml−1) and aged for 24 h. The inset shows a single sunflower assembly. (d) TEM image of sunflower-like hybrid assemblies prepared by subjecting the mixture of PFS30-b-P2VP300seeds and SiO2NPs (as ina) to two heating/cooling cycles (30 and 90 min at 90 °C) followed by aging at room temperature for 24 h. The inset is an image of a single hybrid nanostructure at higher magnification. In the text and theSupplementary Materials, the terms1b,1cand1drefer to the samples whose structures are shown inb–d, respectively. Scale bars, 200 nm and 100 nm in the insets. Figure 1: Preparation of sunflower-like assemblies through seeded growth and self-seeding. ( a ) TEM image of a mixture of SiO 2 NPs and excess PFS 30 - b -P2VP 300 seeds prepared in 2-PrOH and aged for 24 h. ( b ) TEM image of the seed-coated SiO 2 NPs after removal of excess seeds by sedimentation–resuspension in 2-PrOH. The inset shows a single seed-coated SiO 2 NP at higher magnification. ( c ) TEM image of sunflower hybrid assemblies prepared by addition of PFS 30 - b -P2VP 300 in THF (15 μl, 10 mg ml −1 ) to 2-propanol (1 ml) containing seed-coated SiO 2 NPs (0.5 mg ml −1 ) and aged for 24 h. The inset shows a single sunflower assembly. ( d ) TEM image of sunflower-like hybrid assemblies prepared by subjecting the mixture of PFS 30 - b -P2VP 300 seeds and SiO 2 NPs (as in a ) to two heating/cooling cycles (30 and 90 min at 90 °C) followed by aging at room temperature for 24 h. The inset is an image of a single hybrid nanostructure at higher magnification. In the text and the Supplementary Materials , the terms 1b , 1c and 1d refer to the samples whose structures are shown in b – d , respectively. Scale bars, 200 nm and 100 nm in the insets. Full size image A good measure of the control we have over seeded growth is the uniformity of the length of the petal-like micelles that emanate from the central particle. Multiple TEM images were analysed using the software ImageJ, giving a mean petal length L n =224 nm with a narrow distribution (PDI TEM =1.03). Accompanying these sunflower-like structures were occasional isolated linear micelles ( Supplementary Fig. 6 ) with an average length of 547 nm (PDI TEM =1.01). These micelles were most likely nucleated by a few free seed crystallites present in the micelles@SiO 2 NP solution and grew from both ends of the 60nm long seeds. The mean length of the free micelles is approximately twice that of the petals plus the length of the seed. A second processing protocol also leads to the formation of sunflower assemblies. When the solution containing the mixture depicted in Fig. 1a was subjected to two heating–cooling cycles (90 °C, then room temperature) and allowed to age for 24 h, the structures 1d shown in Fig. 1d and Supplementary Fig. 7c,d were obtained. The fibre-like petals of these sunflowers are all similar in length, with L n =204 nm (PDI TEM =1.04). This protocol is conceptually related to ‘self-seeding’ in which heating leads to the selective dissolution of the most soluble crystallites [34] . Upon cooling, the solution becomes supersaturated in BCP, which then deposits epitaxially on the remaining seed crystallites in solution. The disappearance of isolated micelles from the solution indicates that all of the micelles formed upon cooling grew from seeds on the surface of the NPs. It also suggests that adsorption of the seed crystallites on the surface of the SiO 2 NPs suppressed or retarded their dissolution. The sunflower assemblies obtained in this way ( 1d ) appear to be identical to those obtained by seeded growth ( 1c ), except for differences in the lengths of the petals. The two preparation protocols for the construction of sunflower-like hybrid assemblies are summarized in Fig. 2 . 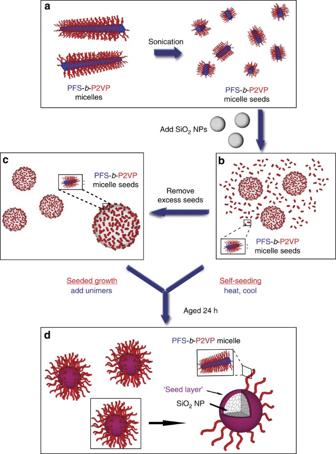Figure 2: Protocols to prepare sunflower-like assemblies. (a) Both strategies begin with sonication of elongated PFS-b-P2VP micelles. (b) Addition of SiO2NPs leads to adsorption of PFS-b-P2VP seed crystallites, but a large excess of seed crystallites remains in solution. (c) In the ‘seeded growth’ strategy, the seed-coated SiO2NPs are first separated from the excess seeds. Then an aliquot of a concentrated solution of PFS-b-P2VP unimers is added, and the mixture is aged to form the mesoscale hybrid structures shown ind. In the ‘self-seeding’ strategy, the mixture inbis annealed at 90 °C, leading to the dissolution of the seed crystallites suspended in solution, but preservation of the crystallites bound to the surface of the SiO2NPs. Upon cooling, micelles grow from the seeds on the NP surface to form hybrid structures indistinguishable from those formed via unimer addition. Both protocols create supersaturated solutions of the BCP in the presence of seed crystallites on the surface of the colloidal nanoparticles, followed by the epitaxial growth of the BCP micelles from the surface-bound seeds. Figure 2: Protocols to prepare sunflower-like assemblies. ( a ) Both strategies begin with sonication of elongated PFS- b -P2VP micelles. ( b ) Addition of SiO 2 NPs leads to adsorption of PFS- b -P2VP seed crystallites, but a large excess of seed crystallites remains in solution. ( c ) In the ‘seeded growth’ strategy, the seed-coated SiO 2 NPs are first separated from the excess seeds. Then an aliquot of a concentrated solution of PFS- b -P2VP unimers is added, and the mixture is aged to form the mesoscale hybrid structures shown in d . In the ‘self-seeding’ strategy, the mixture in b is annealed at 90 °C, leading to the dissolution of the seed crystallites suspended in solution, but preservation of the crystallites bound to the surface of the SiO 2 NPs. Upon cooling, micelles grow from the seeds on the NP surface to form hybrid structures indistinguishable from those formed via unimer addition. Both protocols create supersaturated solutions of the BCP in the presence of seed crystallites on the surface of the colloidal nanoparticles, followed by the epitaxial growth of the BCP micelles from the surface-bound seeds. Full size image Preparation of butterfly-like assemblies The seeded growth protocol can in principle be applied to any type of silica-coated colloidal NPs (for example, metal NPs, quantum dots, magnetic NPs) as the substrate for growing fibre-like micelles. To test this idea, we carried out proof of concept experiments on silica-coated nanorods (NRs) of a nickel–hydrazine complex (SiO 2 @Ni-NRs) reported recently by Gao et al. [35] using them as a template for growing fibre-like micelles from the NR surface. To begin, we synthesized a sample of SiO 2 @Ni-NRs with a mean length L n,rod =375 nm (PDI TEM =1.10) and a silica shell 30 nm thick ( Supplementary Fig. 8a ). Using the same approach described for seeds@SiO 2 NPs, a suspension of SiO 2 @Ni-NRs in 2-PrOH was mixed with PFS 30 - b -P2VP 300 seeds and stirred for 24 h. A TEM image of the as-prepared mixture of SiO 2 @Ni-NRs and seeds is shown in Supplementary Fig. 8b . Most of the unbound excess PFS 30 - b -P2VP 300 seeds were removed by three cycles of sedimentation–resuspension in 2-propanol. The TEM image in Fig. 3a reveals the distinct structure of the SiO 2 @Ni-NRs coated with PFS 30 - b -P2VP 300 seeds ( 3a ). Most of the BCP seeds lie on the NR surface, presumably to maximize hydrogen bonds between the Si-OH groups of the silica and the P2VP corona of the seed micelles. Fewer seeds are attached to the ends of the NRs. 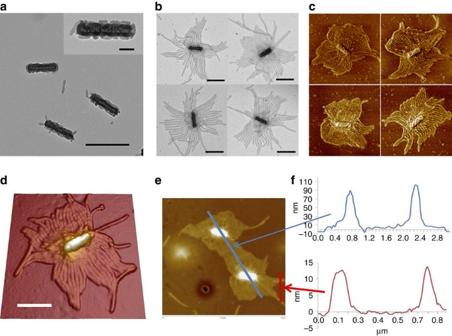Figure 3: Preparation of butterfly-like assemblies through seeded growth. (a) TEM image of PFS30-b-P2VP300seed-coated SiO2@Ni-NRs3aafter removal of the excess PFS30-b-P2VP300crystallites. The inset shows a single seed-coated NR at higher magnification. Scale bar, 500 nm (inset is 100 nm). (b) TEM image of butterfly-like hybrid assemblies. Scale bars, 500 nm.3bprepared by addition of PFS30-b-P2VP300in THF (10 μl, 10 mg ml−1) to 2-propanol (1 ml) containing seed-coated SiO2@Ni-NRs (0.08 mg ml−1) and aged for 24 h. (c) AFM phase images of the butterfly-like hybrid assemblies3b. Each image is 2 × 2 μm. (d) Three-dimensional AFM height image of a single3bassembly. Scale bar, 500 nm. (e) AFM height image (size: 3.5 × 3.5 μm) of two of butterfly-like hybrid assemblies. (f) A section analysis of the two structures inealong the blue and red lines, respectively. The height of the micelle-coated rods is ~\n95 nm, and the height of the micelles themselves is 15 nm. Figure 3: Preparation of butterfly-like assemblies through seeded growth. ( a ) TEM image of PFS 30 - b -P2VP 300 seed-coated SiO 2 @Ni-NRs 3a after removal of the excess PFS 30 - b -P2VP 300 crystallites. The inset shows a single seed-coated NR at higher magnification. Scale bar, 500 nm (inset is 100 nm). ( b ) TEM image of butterfly-like hybrid assemblies. Scale bars, 500 nm. 3b prepared by addition of PFS 30 - b -P2VP 300 in THF (10 μl, 10 mg ml −1 ) to 2-propanol (1 ml) containing seed-coated SiO 2 @Ni-NRs (0.08 mg ml −1 ) and aged for 24 h. ( c ) AFM phase images of the butterfly-like hybrid assemblies 3b . Each image is 2 × 2 μm. ( d ) Three-dimensional AFM height image of a single 3b assembly. Scale bar, 500 nm. ( e ) AFM height image (size: 3.5 × 3.5 μm) of two of butterfly-like hybrid assemblies. ( f ) A section analysis of the two structures in e along the blue and red lines, respectively. The height of the micelle-coated rods is ~\n95 nm, and the height of the micelles themselves is 15 nm. Full size image Seeded growth was carried out by adding an aliquot of PFS 30 - b -P2VP 300 in THF to the suspension of seed-coated NRs in 2-PrOH. Fibre-like micelles grew from the surface of the NRs as shown in Fig. 3b (TEM images) and in Fig. 3c (atomic force microscopy, AFM, phase images) and Fig. 3d (AFM three-dimensional height image). Inspection of these structures ( 3b ) suggests that the fibre-like micelles are primarily oriented perpendicular to the rod axis. This directionality, coupled with the shape of the NR core, is the origin of the butterfly-like shapes of the nanocomposite structures observed on the grid. The micelles were uniform in length ( L n =732 nm, PDI TEM =1.01). A section analysis ( Fig. 3f ) of two adjacent structures in the AFM height image in Fig. 3e shows that the NR cores are ~\n95 nm high, whereas the individual micelles have a height of 15 nm. The nanocomposite structures were accompanied by small numbers of isolated linear micelles that likely originated from seed micelles not attached to the NRs when the THF solution of BCP was added. Control of micelle length From the mechanism of living CDSA, we can anticipate two approaches to control the length of the petal-like micelles in the sunflower hybrid structures. In the first approach, we vary the amount of unimers added to the seeds@SiO 2 NPs as shown as pathway c→d in Fig. 2 . If all the seeds initiate micelle growth simultaneously and the micelles grow at the same rate, then the length of the petals should depend upon the ratio of unimers added to seeds present on the surface of the NPs. We demonstrate this idea in Fig. 4a,b (and Supplementary Figs 9 and 10 ), where we compare TEM images of hybrid structures obtained by adding two different amounts of PFS 30 - b -P2VP 300 (10 mg ml −1 in THF) to portions of a solution of 1b (seeds@SiO 2 NPs) in 2-PrOH. Analysis of the micelle lengths in the micrographs indicated that the lengths obtained with the 10 μl addition of unimer ( 4a , L n =366 nm, PDI TEM =1.04) was approximately half that of 20 μl addition ( 4b , L n =704 nm, PDI TEM =1.01). 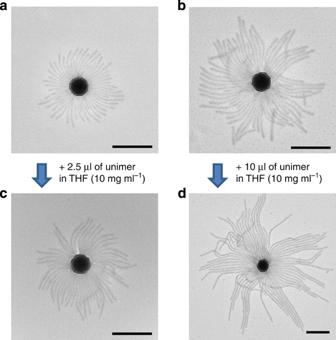Figure 4: Controlling micelle length in hybrid constructions. TEM images of the structures obtained by adding different amounts (a, 10 μl orb, 20 μl) of PFS30-b-P2VP300in THF (10 mg ml−1) to 2-PrOH solutions (1 ml) of seed-coated SiO2NPs (0.25 mg), then aging 24 h at room temperature. (c) Two-step micelle growth. Hybrid sunflower structures4cwith elongated petals obtained by adding an aliquot of PFS30-b-P2VP300in THF (2.5 μl, 10 mg ml−1) to a 2-PrOH solution (0.5 ml) of the sunflower assemblies4ashown ina. (d) Larger structures4dobtained by adding PFS30-b-P2VP300in THF (10 μl, 10 mg ml−1) to a 2-PrOH solution (0.5 ml) of the assemblies4bshown inb. Both solutions were aged for 24 h after the second addition of PFS30-b-P2VP300. Scale bars, 500 nm. Figure 4: Controlling micelle length in hybrid constructions. TEM images of the structures obtained by adding different amounts ( a , 10 μl or b , 20 μl) of PFS 30 - b -P2VP 300 in THF (10 mg ml −1 ) to 2-PrOH solutions (1 ml) of seed-coated SiO 2 NPs (0.25 mg), then aging 24 h at room temperature. ( c ) Two-step micelle growth. Hybrid sunflower structures 4c with elongated petals obtained by adding an aliquot of PFS 30 - b -P2VP 300 in THF (2.5 μl, 10 mg ml −1 ) to a 2-PrOH solution (0.5 ml) of the sunflower assemblies 4a shown in a . ( d ) Larger structures 4d obtained by adding PFS 30 - b -P2VP 300 in THF (10 μl, 10 mg ml −1 ) to a 2-PrOH solution (0.5 ml) of the assemblies 4b shown in b . Both solutions were aged for 24 h after the second addition of PFS 30 - b -P2VP 300 . Scale bars, 500 nm. Full size image The second approach involves sequential addition of BCP to preformed mesostructures. Here we added 2.5 μl PFS 30 - b -P2VP 300 in THF to an aliquot of solution 4a and 10 μl to an aliquot of solution 4b . After 24 h aging, we found that the 366nm petals of 4a ( Fig. 4a ) grew to 510 nm ( 4c , PDI TEM =1.02, Fig. 4c and Supplementary Fig. 11 ), and from 704 nm ( 4b , Fig. 4b ) to 1.36 μm ( 4d , PDI TEM =1.01, Fig. 4d and Supplementary Fig. 12 ). These experiments demonstrate that the end of the petals were still active for further growth. Further functionalization of the hybrid structures The sequential addition of BCP for petal elongation opens the possibility for constructing many new types of structures through site-specific placement of different corona chains in the micelles emanating from the NP surface. As a proof of concept, we show, based on an idea in ref. 36 , how one can attach cationic charges to the tips of the micelles as means of introducing small metal NPs [36] . To introduce these cationic sites, we took a sample of PFS 30 - b -P2VP 300 and partially quaternized the pyridines with methyl iodide (PFS 30 - b -P2VP 300 Q ). The challenge that we faced here was to keep the extent of methylation small (~\n3%) to maintain polymer solubility in THF. At this level of methylation, each P2VP chain contains only ~\n10 positively charged pyridinium groups. When we added a THF solution of the partially quaternized polymer (PFS 30 - b -P2VP 300 Q , 2.5 μl, 10 mg ml −1 ) to 0.5 ml aliquots of 4a and 4b in 2-PrOH, we obtained the structures shown, respectively, in Fig. 5a,d . As one might expect, there is insufficient contrast to see the location of the newly added polymer. We note that the average petal lengths of the two sets of structures increased from L n =366nm in 4a to 502 nm in 5a (PDI TEM =1.02, Fig. 5a ), and from L n =704nm in 4b to 853 nm in 5d (PDI TEM =1.01, Fig. 5d ), introducing sites of positive charge in the distal part of each petal. 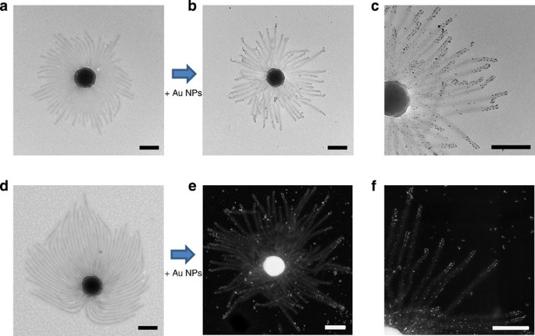Figure 5: Sunflower-like assemblies with partially functionalized petals. (a) TEM image of sample5aobtained by the addition of the partially quaternized block copolymer PFS30-b-P2VP300Qto4ain 2-PrOH. (d) TEM image of sample5dobtained by addition of PFS30-b-P2VP300Qto4bin 2-PrOH. Both solutions were aged for 24 h at room temperature. (b,e) Treatment of5aand5din 1:1 2-PrOH/H2O with negatively charged Au NPs, led to the structures5b(b) and5e(dark-field TEM image,e, respectively. (c) Higher magnification image from a different position of the same grid used to obtain the image inb. (f) Higher magnification image from a different position of the same grid used to obtain the image ine. Scale bars, 250 nm. Figure 5: Sunflower-like assemblies with partially functionalized petals. ( a ) TEM image of sample 5a obtained by the addition of the partially quaternized block copolymer PFS 30 - b -P2VP 300 Q to 4a in 2-PrOH. ( d ) TEM image of sample 5d obtained by addition of PFS 30 - b -P2VP 300 Q to 4b in 2-PrOH. Both solutions were aged for 24 h at room temperature. ( b , e ) Treatment of 5a and 5d in 1:1 2-PrOH/H 2 O with negatively charged Au NPs, led to the structures 5b ( b ) and 5e (dark-field TEM image, e , respectively. ( c ) Higher magnification image from a different position of the same grid used to obtain the image in b . ( f ) Higher magnification image from a different position of the same grid used to obtain the image in e . Scale bars, 250 nm. Full size image To map the location of the cationic charges in the elongated micelles, we treated the suspensions of mesostructures 5a and 5d in 2-PrOH/H 2 O (1:1 (v/v)) with negatively charged 2-nm gold NPs (Au NPs bearing mercaptoacetate surface groups) and obtained colloidally stable solutions of the structures 5b ( Fig. 5b ) and 5e ( Fig. 5e ), respectively. There is a clear indication, especially in high magnification images (TEM Fig. 5c , and dark-field TEM Fig. 5f ), of the preferential attachment of the Au NPs to the ends of the petals where the partially quaternized polymer was located. More important, these experiments demonstrate that the hybrid mesostructures maintain their integrity over the course of these modifications. They also suggest that it is possible to introduce a variety of different inorganic NPs at specific locations along the micelles. In summary, we have demonstrated a new and versatile approach to fabricate colloidal mesoscale hybrid assemblies consisting of brushes of cylindrical BCP micelles attached to the surface of silica-coated NPs of arbitrary shape. The key step in the fabrication design was to attach seed crystallites of the BCP micelles to the NP surface followed by CDSA of added BCP. In this way, core-crystalline micelles grow from the NP surface. In the case where the newly added polymer carried positive charges in the corona, its locus in the brush could be further functionalized by selective adsorption of negatively charged Au NPs. This procedure also demonstrates that the hybrid mesostructures are sufficiently robust to be post-modified. Although the specific proof of concept example described here involved PFS 30 - b -P2VP 300 as the micelle forming polymer, the fabrication protocol should in principle apply to any BCP that forms elongated core-crystalline micelles and to any substrate to which the corona chains of the seed crystallites can attach. For example, we have recently shown that CDSA can be extended to BCP micelles with a conjugated crystalline polythiophene core [22] , [37] . An interesting system for future studies would be hybrids consisting of polythiophene BCP micelles and titanium oxide NPs to generate potential light harvesting photovoltaic structures. Thus we anticipate that a broad variety of novel, interesting and ultimately functional mesostructures can be created in this way. Materials Tetrahydrofuran (THF, ACS reagent, ≥99.0%), isopropanol (2-PrOH, ≥99.5%), hexane (≥99.8%), tetraethyl orthosilicate (TEOS, ≥99.0%), didodecyldimethylammonium bromide (DDAB, 98%), mercaptoacetic acid (≥98%), Brij 58, diethylamine (≥99.5%), hydrazine hydrate (reagent grade, 50–60%), nickel dichloride (NiCl 2 , 98%), dodecylamine (≥99%), gold(III) chloride (AuCl 3 , 99%), TBAB (tetra- n -butylammonium bromide, ≥98%), tetramethylammonium hydroxide (Me 4 N + [OH] − , 10% in water) were purchased from Sigma-Aldrich and used as received. PFS 30 - b -P2VP 300 ( M n,GPC =30,400, PDI=1.17) is the same sample reported in ref. 32 , and was synthesized by He et al. by sequential anionic polymerization. Electron microscopy Bright-field transmission electron microscopy (TEM) images were taken using a Hitachi H-7000 instrument. For each sample, micelle length distributions were determined by tracing more than 100 individual micelles or corona micelles grown from NPs or NRs using the software ImageJ (NIH, US). Dark-field TEM images were taken using a FEI QUANTA model FEG 250 ESEM with a BF/DF STEM detector in the high vacuum mode with an accelerating voltage of 30 kV. Scanning electron microscopy (SEM) images were taken using a Hitachi S-5200 SEM instrument. Energy-dispersive X-ray spectroscopy (EDX) analysis for PFS- b -P2VP unimers or seed-coated silica NPs were taken using an EDX attachment (INCA, Oxford Instruments) on the Hitachi S-5200 SEM instrument. Composition-based line scans were carried out on relevant particles identified on the sample grid. The accelerating voltage for EDX measurements was 15 kV, and the current was 20 μA. Data were collected over a period of 5 min. EDX was used to determine the incorporation of PFS- b -P2VP copolymers or seeds onto the surface of silica NPs. Samples were prepared by placing one drop of solution on a Formvar-carbon coated grid, touching the edge of the droplet with a filter paper to remove excess liquid and allowing the grid to dry. The number average lengths ( L n ) and weight average lengths ( L w ) of the micelles were calculated from the TEM images by tracing by hand more than 100 individual micelles or corona micelles using the software ImageJ (NIH, US). Values of L n and L w were calculated as where N i is the number of micelles of length L i , and N is the total number of micelles examined for each sample. The distribution of micelle lengths (PDI TEM ) is characterized by L w / L n . The number and weight average diameters of the silica NPs ( d n , d w ), the number average lengths ( L n,rod , L w,rod ) and the average widths ( W n,rod , W w,rod ) of the silica-coated nickel–hydrazine complex, and the average thicknesses ( T n , T w ) of the silica layer or polymer layer and their distributions were calculated in a similar way. Atomic force microscopy AFM measurements were carried out with an instrument (Digital Instruments, Dimension 5000, Nanoscope IIIa, US) using the same samples prepared for TEM. High resonance frequency silicon probes with spring constant 42 N m −1 , resonance frequency ~\n320 kHz, (NanoWorld, Switzerland) were used for tapping-mode imaging in air. The scan rate was 1 Hz and the collected images were 512 pixels × 512 pixels. Height and phase images were analysed by software (Nanoscope V1.40). Dynamic light scattering The hydrodynamic diameters and polydispersity index (PDI) of silica NPs in THF or 2-PrOH, silica NPs mixed with PFS- b -P2VP unimers in THF and silica NPs mixed with PFS- b -P2VP seeds in 2-PrOH ( Supplementary Table 1 ) were determined with a BI-90 particle sizer (Brookhaven Instruments Corporation, Holtsville, NY). For some selected samples, the autocorrelation and CONTIN plots of the sunflower hybrid assembly ( Supplementary Fig. 10e,f ) were obtained using an ALV/ DLS/SLS-5000 Compact Goniometry System equipped with a vertically polarized He–Ne laser ( λ 0 =632.8 nm, 35 mW) as the light source and a Dual ALV-High Q.E. APD avalanche photodiode module connected to an ALV-5000/EPP multiple digital time correlator as the detection module. The experiments were performed at 90°. For the measurement, the sample was sealed in a screw-capped vial and immersed in a toluene vat which matched the index of refraction of the glass vial. Partially quaternized PFS 30 - b -P2VP 300 Q The partially quaternized PFS 30 - b -P2VP 300 copolymer was prepared following the protocol described in ref. 36 . Cylindrical micelles were first prepared by dissolving PFS 30 - b -P2VP 300 (5 mg) in THF (100 μl), adding this solution to 2-PrOH (5 ml), and setting it aside to age for 24 h. This sample was briefly sonicated using a 70W ultrasonic bath to shorten the length of the micelles. To this solution (5.0 mg per 5 ml, pyridyl group content: 4.9 × 10 −2 mmol) was added MeI (3.0 μl, 4.9 × 10 −2 mmol) at room temperature with stirring. After 24 h, the solvent was evaporated, and the product was purified by dissolution in THF followed by precipitation and washing with hexane. This cycle was repeated three times and the partially quaternized polymer was dried under vacuum at room temperature for 2 days. The degree of quaternization was evaluated by 1 H NMR in d 6 -dimethylsulphoxide, noting that after quaternization, the chemical shift of the α-H in pyridine ring shifted from 8.26 to 8.67 p.p.m. A degree of quaternization of ~\n3.2% was determined by comparing the integrated 1 H NMR signals of the shifted α-H peak at 8.67 p.p.m. to that of the α-H peak at 8.26 p.p.m. in the pyridine ring. Gold nanoparticles coated with 2-mercaptoacetic acid Au NPs were synthesized following the procedure described in ref. 36 . Briefly, DDAB was dissolved in toluene to make a 100 mM stock solution. Gold(III) chloride (AuCl 3 , 7.5 mg) was dissolved by sonication in the DDAB solution (2.5 ml) leading to an orange-red colour. Dodecylamine (18 mg) was dissolved in 0.5 ml of the DDAB solution by sonication and added to the solution containing AuCl 3 . In another vial TBAB (25 mg) was dissolved in 1 ml of the DDAB solution and injected into the gold salt solution under vigorous stirring at room temperature. The colour of the solution turned dark brown immediately suggesting the formation of Au NPs. To perform ligand exchange with mercaptoacetic acid, 1 ml of methanol was added to the Au NP solution (0.5 ml). The NPs precipitated immediately, were collected by centrifugation, and then redispersed in 0.5 ml of toluene. To this solution was added about 10 mg of mercaptoacetic acid. The Au NPs precipitated immediately and were collected by centrifugation. After washing the precipitate with toluene (1 × 1 ml), methanol (3 × 1 ml) and water (3 × 1 ml), the Au NPs were redispersed in 0.5 ml water containing sufficient 10% aqueous solution of Me 4 N + [OH] − to raise the pH to 10. By TEM, the mean diameter of the Au NPs was ~\n2 nm. Preparation of PFS- b -P2VP seed crystallites PFS 30 - b -P2VP 300 seed crystallites were prepared in two steps. First, long micelles were prepared by dissolving the polymer (1 mg) in THF (100 μl), adding this solution to 2-PrOH (2 ml), and setting it aside to age for 24 h. This mixture was then sonicated at room temperature for three 10-min periods using a 70W ultrasonic bath. The micelle seed fragments obtained ( L n =60 nm, PDI TEM =1.09) were characterized by measuring over 200 seeds in several TEM images. Preparation of silica nanoparticles (SiO 2 NPs) Silica NPs (SiO 2 NPs) were prepared by a modified Stöber method as described in ref. 38 . Briefly, TEOS (9 ml) was slowly added to a mixture of ethanol (150 ml), deionized water (15 ml), and aqueous ammonia (27%, 3 ml) at room temperature. The mixture was stirred vigorously for 24 h. The SiO 2 NPs were purified by three sedimentation–resuspension cycles in a 1:1 ethanol:deionized water mixture. Finally, a dried powder of NPs (SiO 2 NPs) was obtained by freeze-drying over 24 h. The number average diameter ( d n ) of the SiO 2 NPs was 246 nm, PDI TEM =1.01, evaluated by measuring over 100 SiO 2 NPs in several TEM images. Preparation of SiO 2 @Ni-NRs The silica-coated nickel–hydrazine complex NRs (SiO 2 @Ni-NRs) were synthesized following the procedure described in ref. 35 . Brij 58 (8.5 g) was dissolved in cyclohexane (15 ml) at 50 °C. Then, a NiCl 2 solution in water (1.7 ml, 0.1 g ml −1 ) was added and stirred until a homogeneous solution was obtained. Hydrazine hydrate (0.45 ml) was added dropwise. The mixture was stirred for 3 h. Then, diethylamine (1 ml) and subsequently TEOS (3 ml) were added to the system. The silica coating process was allowed to proceed for 2 h, followed by centrifugation and washing with ethanol (40 ml, three times) and 2-PrOH (40 ml, three times). Finally, the SiO 2 @Ni-NRs were dispersed in 2-PrOH (25 ml) as a stock solution for further experiments. The solids concentration was 32.2 mg ml −1 . The number average length ( L n,rod ) of the SiO 2 @Ni-NRs was 375 nm (PDI TEM =1.01), with a number average width ( W n,rod ) of 93 nm (PDI=1.06); the number average thickness ( T n ) of the silica layer was 30 nm (PDI TEM =1.03). These values were evaluated by measuring over 100 NRs ( L n,rod ) or 100 positions along the rods ( W n,rod , T n ) in several TEM images. Preparation of PFS- b -P2VP seed-coated NPs 1b and 3a Two kinds of PFS 30 - b -P2VP 300 seed-coated NPs (SiO 2 NPs or SiO 2 @Ni-NRs) were prepared by the same procedure. For structures 1b , a sample of SiO 2 NPs (1 mg) was dispersed in 2-PrOH (1 ml), followed by the addition of a 2-PrOH solution (1 ml) containing PFS 30 - b -P2VP 300 seeds (0.5 mg, L n =60 nm). The mixture was stirred 24 h, and a drop of the solution was taken for TEM image analysis ( Fig. 1a and Supplementary Fig. 3 ). Excess seeds were removed by three sedimentation–resuspension cycles. As part of each resuspension step, the samples were sonicated briefly (~\n2 s) in a 70W ultrasonic bath. Finally, the PFS 30 - b -P2VP 300 seed-coated SiO 2 NPs were redispersed in 2-PrOH (2 ml) for TEM image analysis ( Fig. 1b and Supplementary Fig. 4 ). An EDX line scan showing strong signals for Fe and N is presented in Supplementary Fig. 5 . An EDX line scan of the precursor SiO 2 NPs shows no signal for Fe ( Supplementary Fig. 13 ) or N (not shown). Structures 3a were prepared by the same method. A 2-PrOH solution (1 ml) containing PFS 30 - b -P2VP 300 seeds (0.15 mg, L n =60 nm) was mixed with a 2-PrOH solution (1 ml) containing dispersed SiO 2 @Ni-NRs (0.16 mg). The mixture was stirred 24 h, and a drop of the solution was taken for TEM image analysis. Excess seeds were removed by three sedimentation–resuspension cycles, and the samples were sonicated briefly during each resuspension step. Finally, the PFS 30 - b -P2VP 300 seed-coated SiO 2 @Ni-NRs were redispersed in 2-PrOH (2 ml). Coating SiO 2 NPs with PFS- b -P2VP unimers in THF A sample of SiO 2 NPs (1 mg) dispersed in THF was treated with a solution of PFS 30 - b -P2VP 300 (THF, 1 mg, 2 ml), stirred 24 h, purified by sedimentation–redispersion, and examined by TEM and EDX spectroscopy. EDX line scan analysis of these SiO 2 NPs ( Supplementary Fig. 14 ) showed small Fe and N peaks, indicating the presence of a very thin film of BCP on the surface of the SiO 2 NPs. These particles were then transferred to 2-PrOH and treated with a solution of PFS 30 - b -P2VP 300 in THF (80 μl, 10 mg ml −1 ) in an attempt to induce the growth of PFS 30 - b -P2VP 300 micelles from the surface of the NPs. TEM images taken after 24 h ( Supplementary Fig. 15 ) showed a superposition of long fibre-like BCP micelles and isolated silica NPs. Both species remained colloidally stable upon aging for several days. Preparation of samples 1c and 3b by seeded growth For micelles@SiO 2 NPs ( 1c ), an aliquot of PFS 30 - b -P2VP 300 in THF (15 μl, 10 mg ml −1 ) was added to a 2-PrOH solution (1 ml) containing PFS 30 - b -P2VP 300 seed-coated SiO 2 NPs (0.5 mg of SiO 2 NPs purified to remove excess of PFS 30 - b -P2VP 300 seeds). After brief swirling, the solution was allowed to age for 24 h. Humidity affected the appearance of the self-assembled structures: when the sample was deposited on the TEM grid on a humid day, the micelle petals of the sunflower assemblies tended to stick together (see Supplementary Fig. 16 ). To eliminate the effect of humidity on sample preparation for TEM imaging, we prepared all TEM samples in a glove bag under a dry nitrogen atmosphere. To grow micelles from the surface of SiO 2 @Ni-NRs, an aliquot of PFS 30 - b -P2VP 300 in THF (10 μl, 10 mg ml −1 ) was added to a 2-PrOH solution (1 ml) containing seed-coated SiO 2 @Ni-NRs (0.08 mg of SiO 2 @Ni-NRs purified to remove excess seeds). After brief swirling, the solution was allowed to age for 24 h. Preparation of sample 1d by self-seeding A 2-PrOH solution (2 ml) containing a mixture of SiO 2 NPs (1 mg) and PFS 30 - b -P2VP 300 seeds (0.8 mg) was subjected to two successive heating/cooling cycles. The solution was first heated at 90 °C for 30 min, cooled to room temperature, and then aged for 24 h. A drop of the sample was taken out for TEM image analysis. The remaining solution was re-heated at 90 °C for 90 min, cooled to room temperature, and aged for another 24 h before aliquots were taken for analysis by TEM. Controlling petal length of samples 4a and 4b An aliquot of a 2-PrOH stock solution (1 ml) containing PFS 30 - b -P2VP 300 seed-coated SiO 2 NPs (0.5 mg) was diluted with 2-PrOH (1 ml), and divided into two portions. To one portion, an aliquot of PFS 30 - b -P2VP 300 in THF (10 μl, 10 mg ml −1 ) was added. The mixture was swirled briefly and then aged for 24 h. A TEM image of the structures obtained ( L n =366 nm, PDI TEM =1.04) are shown in Fig. 4a and Supplementary Fig. 9 . We refer to this sample as sunflower 4a . To the second portion of seed solution a larger aliquot of PFS 30 - b -P2VP 300 in THF (20 μl, 10 mg ml −1 ) was added. The mixture was swirled briefly and then aged for 24 h. A TEM image of the structures obtained ( L n =704 nm, PDI TEM =1.01) are shown in Fig. 4b and Supplementary Fig. 10 . We refer to this sample as sunflower 4b . Petal elongation of samples 4c and 4d The sunflower hybrids 4a and 4b were used as starting materials for a second stage of seeded growth. After aging these samples for 2 days, they were treated with additional amounts (2.5 μl for 4a , 10 μl for 4b ) of PFS 30 - b -P2VP 300 in THF (10 mg ml −1 ). The mixtures were swirled for a few seconds and aged for 24 h before aliquots were taken for analysis by TEM. Representative images are presented in Fig. 4c,d and Supplementary Figs. 11 and 12 . For petal elongation with PFS 30 - b -P2VP 300 Q ( 5a and 5d ) and selective functionalization of the quaternized segments with Au NPs ( 5b,c and 5e,f ), samples of sunflower hybrids 4a and 4b were each treated with a solution of PFS 30 - b -P2VP 300 Q in THF (2.5 μl, 10 mg ml −1 ). The mixtures were swirled briefly and then aged for 24 h. TEM images of the sunflower structures obtained in this way are shown in Fig. 5a (from sample 4a ) and Fig. 5d (from sample 4b ). To attach Au NPs to the quaternized segments, a sample of this solution (50 μl) was diluted with an equal volume of water. Separately, a sample of negatively charged Au NPs was dispersed in water and treated with Me 4 N + OH − (10% in water) to bring the pH to 10 and the Au NP concentration to ~\n4 mM). Then 4 μl of this solution was added to the 100μl sunflower block comicelle solution, swirled briefly and allowed to age for 3 h before grids were prepared for bright-field and dark-field TEM analysis. How to cite this article: Jia, L. et al. A design strategy for the hierarchical fabrication of colloidal hybrid mesostructures. Nat. Commun. 5:3882 doi: 10.1038/ncomms4882 (2014).